Distinct bone marrow-derived and tissue-resident macrophage lineages proliferate at key stages during inflammation The general paradigm is that monocytes are recruited to sites of inflammation and terminally differentiate into macrophages. There has been no demonstration of proliferation of peripherally-derived inflammatory macrophages under physiological conditions. Here we show that proliferation of both bone marrow-derived inflammatory and tissue-resident macrophage lineage branches is a key feature of the inflammatory process with major implications for the mechanisms underlying recovery from inflammation. Both macrophage lineage branches are dependent on M-CSF during inflammation, and thus the potential for therapeutic interventions is marked. Furthermore, these observations are independent of Th2 immunity. These studies indicate that the proliferation of distinct macrophage populations provides a general mechanism for macrophage expansion at key stages during inflammation, and separate control mechanisms are implicated. Monocytic cells have fundamental roles in both tissue homoeostasis and immune regulation where they influence the initiation and resolution of inflammation. To support these activities, monocytes and macrophages exhibit distinct effector functions and display a high degree of heterogeneity [1] , [2] . Human subsets of blood monocytes are distinguished by their expression of CD14 and CD16 (ref. 3 ). Similarly in mice, monocyte subsets are separated by expression of CCR2, Ly-6C, CD62L, CX 3 CR1, CD43 and Ly-6B.2 (7/4 antigen) [4] , [5] , [6] . These monocyte subsets have been classified as ‘classical’, ‘intermediate’ and ‘non-classical’ [7] . During inflammation, the generally accepted model is one where monocytes are recruited to inflammatory lesions, whereupon they mediate various effector functions and differentiate into macrophages and dendritic cells [1] , [2] , [4] , [8] , [9] , [10] . It is, however, unclear how these various populations govern their numbers and activities to ensure both competent host defence and the restoration of normal tissue homoeostasis. The bulk of recruited monocytes appear to be of the ‘classical’ subset recruited though a CCR2-mediated process [4] , [8] . In mice, these classical monocytes are also labelled with the Ly-6B.2 antigen (simplified henceforth to Ly-6B) [6] , [11] , [12] , a marker, which appears to be retained for some time (>14 h based on adoptive transfer experiments) on newly differentiated macrophages within inflammatory lesions [11] , [12] . These monocytic populations are quite distinct from tissue-resident (Res) macrophages, which contribute to the initiation of inflammation, but also serve to maintain tissue homoeostasis via surveillance of local microenvironment [2] , [13] . In several tissues, including serosal tissues such as the peritoneal cavity, Res macrophage numbers are rapidly lost following the initiation of inflammation in a response referred to as the ‘disappearance reaction’ [14] . The disappearance reaction has been attributed to increased adherence to structural tissues, increased cell death or emigration to draining lymph nodes [14] . This disappearance is akin to the loss of Langerhans cells from the epidermis [15] and alveolar macrophages from the lung [16] , [17] during inflammation. However, as inflammation proceeds, cells displaying a characteristic Res macrophage phenotype reappear in the presence of ‘inflammation-associated’ macrophages [6] , [18] , [19] through proliferation of residual mature Res macrophages that survived the inflammatory process. These Res macrophages appear capable of self-renewal with little input from the peripheral monocyte pool [13] , [18] , indicating that they represent a distinct branch in the lineage. Indeed, postnatal development of peritoneal Res macrophages also appears to occur by proliferation [13] , [18] . These results are consistent with the development and expansion of Langerhans cells in the skin [20] , [21] and microglia in the brain [22] , [23] . Identification of this self-renewal mechanism adds a new layer of complexity to the classical model of monocyte to macrophage differentiation and led us to re-evaluate the control of macrophage turnover during inflammation. In the peritoneal cavity, Res macrophages are characterized by an F4/80 high CD11b high phenotype that distinguishes them not only from other tissue-resident phagocytes [18] , [19] , [24] but also from inflammatory monocytes and macrophages that broadly express lower levels of F4/80 (refs 6 , 12 , 25 ). We show that these subsets are not terminally differentiated and instead continue to actively proliferate at distinct stages during the resolution of an inflammatory response. As well as proliferation of Res macrophages, this includes a distinct lineage of recruited bone marrow (BM)-derived macrophages that proliferate within the inflammatory lesion. As a consequence, our data change our understanding of monocyte/macrophage biology by emphasizing that proliferative mechanisms, in addition to chemokine-directed trafficking, contribute to the turnover of monocytic cells at sites of inflammation. Characterization of Ly-6B-positive inflammatory macrophages Zymosan-induced peritonitis triggers a rapid, but transient elevation in neutrophil numbers and is followed by a more protracted elevation in eosinophil numbers ( Fig. 1a , left). At the same time, we observed a rapid drop in total monocyte/macrophage numbers, caused by the loss of F4/80 high Res macrophages. This is followed by a rapid influx of peripheral inflammatory monocytes/macrophages and a slower return of Res macrophages, identified by their F4/80 high CD11b high phenotype [18] ( Fig. 1a , right). The phenotype of the inflammatory macrophage infiltrate is heterogeneous and Ly-6B + inflammatory macrophages are clearly evident from day 2 of inflammation. The Ly-6B + inflammatory macrophages are present throughout the resolution phase of inflammation and are still detectable at 14 days after zymosan administration ( Fig. 1b ). Examination of macrophage populations in a higher dose zymosan model (2 × 10 7 particles intraperitoneally (i.p.)) and an alternate thioglycollate peritonitis model showed similarities and differences ( Fig. 1d ). The higher dose zymosan model was characterized by lower number of Res macrophages ( Fig. 1d , middle) when compared with the low dose model ( Fig. 1d , left). This difference likely reflects the more substantial inflammatory burden, which may ultimately delay the resolution of inflammation. The thioglycollate model, which is characterized by substantial inflammation and a large accumulation of inflammatory macrophages, showed little evidence of resolution at this time point (as indicated by the number of Res macrophages) and notably no significant evidence of peritoneal Ly-6B-expressing inflammatory macrophages. Ly-6B-expressing macrophages were purified by flow-cytometric sorting and found to have a size and morphology consistent with macrophages ( Fig. 1e ). 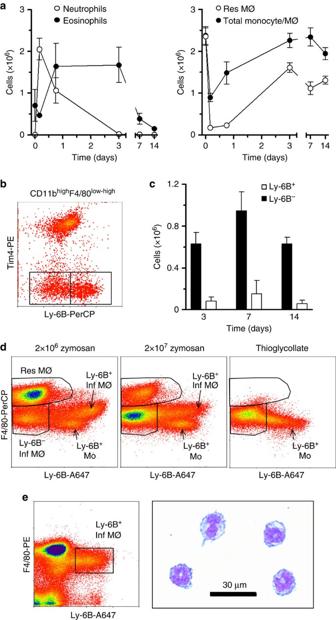Figure 1: Kinetics of acute zymosan-induced peritonitis and appearance of Ly-6B-expressing inflammatory macrophages (MØ). (a) Graphs showing the numbers of neutrophils and eosinophils (left panel) and MØ (both total monocyte/MØ and Res MØ) MØ (right panel) present at the indicated times after i.p. administration of 2 × 106zymosan particles. Data represent mean±s.e.m. of 3–5 individual mice per time point, taken from one of two similar experiments. (b) Representative flow-cytometric profiles showing Ly-6B+inflammatory (Inf) MØ, identified as previously described6,18by gating on CD11bhighF4/80low-highcells (excluding eosinophils), are clearly distinct from Tim4highRes MØ. Gates denote Ly-6B+and Ly-6B−Inf MØ populations. (c) Approximately a fifth of cells classified as Inf MØ are Ly-6B+and are present for several weeks after induction of a mild inflammatory reaction. Data are taken from the animals represented in panelaabove and presented as mean±s.e.m. (d) Representative flow-cytometric profiles (gated on F4/80low-highCD11b+monocytes and MØ) taken from mice 72 h after induction of peritonitis with zymosan (both 2 × 106and 2 × 107particles) and thioglycollate broth, as indicated. The higher dose of zymosan resulted in similar MØ populations, but with substantially reduced recoverable numbers of Res MØ when compared with the low dose, as expected12,25. In contrast, thioglycollate broth resulted in a near complete depletion of Res MØ and no evident Ly-6B+Inf MØ population at this time. The presence of both Ly-6B+monocytes and Ly-6B+Inf MØ populations are indicated. Flow-cytometric plots are representative of at least three mice per group from one of two similar experiments. (e) The Ly-6B-expressing MØ were gated as indicated (left panel) and purified (>90%) by flow-cytometric cell sorting and analysed on cytospins stained with eosin and methylene blue. Cells were pooled from 6-week-old female C57BL/6 mice 7 days after i.p. zymosan (2 × 106particles). Figure 1: Kinetics of acute zymosan-induced peritonitis and appearance of Ly-6B-expressing inflammatory macrophages (MØ). ( a ) Graphs showing the numbers of neutrophils and eosinophils (left panel) and MØ (both total monocyte/MØ and Res MØ) MØ (right panel) present at the indicated times after i.p. administration of 2 × 10 6 zymosan particles. Data represent mean±s.e.m. of 3–5 individual mice per time point, taken from one of two similar experiments. ( b ) Representative flow-cytometric profiles showing Ly-6B + inflammatory (Inf) MØ, identified as previously described [6] , [18] by gating on CD11b high F4/80 low-high cells (excluding eosinophils), are clearly distinct from Tim4 high Res MØ. Gates denote Ly-6B + and Ly-6B − Inf MØ populations. ( c ) Approximately a fifth of cells classified as Inf MØ are Ly-6B + and are present for several weeks after induction of a mild inflammatory reaction. Data are taken from the animals represented in panel a above and presented as mean±s.e.m. ( d ) Representative flow-cytometric profiles (gated on F4/80 low-high CD11b + monocytes and MØ) taken from mice 72 h after induction of peritonitis with zymosan (both 2 × 10 6 and 2 × 10 7 particles) and thioglycollate broth, as indicated. The higher dose of zymosan resulted in similar MØ populations, but with substantially reduced recoverable numbers of Res MØ when compared with the low dose, as expected [12] , [25] . In contrast, thioglycollate broth resulted in a near complete depletion of Res MØ and no evident Ly-6B + Inf MØ population at this time. The presence of both Ly-6B + monocytes and Ly-6B + Inf MØ populations are indicated. Flow-cytometric plots are representative of at least three mice per group from one of two similar experiments. ( e ) The Ly-6B-expressing MØ were gated as indicated (left panel) and purified (>90%) by flow-cytometric cell sorting and analysed on cytospins stained with eosin and methylene blue. Cells were pooled from 6-week-old female C57BL/6 mice 7 days after i.p. zymosan (2 × 10 6 particles). Full size image Inflammatory macrophages are bone-marrow derived We have classified inflammatory macrophages as those ‘associated with inflammation’, but without definitively ascribing their origins to distinguish them from tissue-resident cells (this article and Davies et al. [18] ). Adoptive transfer experiments designed to track the persistence of resident peritoneal cells during an acute inflammatory episode indicated that inflammatory macrophages, including the Ly-6B-expressing cells, were not initially present in the peritoneal cavity [18] . We addressed the issue of the origins of Ly-6B + and Ly-6B − inflammatory macrophages directly, with partial BM chimeras created by shielding the peritoneal cavity before irradiation and reconstitution with CD45-mismatched BM (CD45.2 + donor cells into CD45.1 + recipients) [26] . After 6 weeks, the partial chimerism was confirmed by analysis of the myeloid cells in peripheral blood ( Fig. 2a ). Zymosan peritonitis was induced in the partial chimeras, exactly as described [18] , and then at day 3 the principle subsets of macrophages under study were gated as shown ( Fig. 2b ). Consistent with the direct evidence from previous adoptive transfer experiments in this model [18] , the Res macrophages remained of recipient origin, but both the Ly-6B + and Ly-6B − inflammatory macrophages were chimeric ( Fig. 2c ). When quantified in individual chimeras, there was a clear correlation between blood monocyte chimerism and inflammatory macrophage chimerism demonstrating that the Ly-6B + inflammatory macrophages were BM derived ( Fig. 2d ). 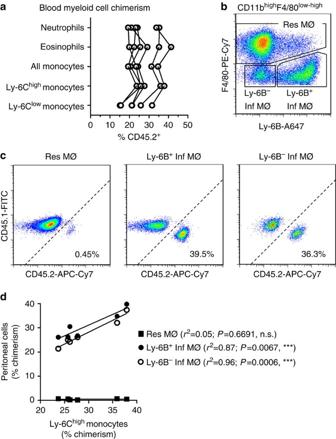Figure 2: Both Ly-6B+and Ly-6B−inflammatory macrophages (MØ) are derived from the bone marrow. Partial BM chimeras were generated as previously described26, after shielding the peritoneal cavity, and then were left to recover for 6 weeks. (a) Analysis of blood myeloid cell chimerism 1 day before induction of peritonitis shows a stable chimerism in all experimental animals. Each line links the data from an individual mouse. (b) Gating strategy for the identification of Res and inflammatory (Inf) MØ (both Ly-6B+and Ly-6B−) 72 h after the induction of peritonitis by i.p. administration of 2 × 106zymosan particles. The plot has been pre-gated on CD11bhighF4/80low-highcells as previously reported18. (c) Representative flow-cytometric analysis of the indicated MØ subsets to determine the level of chimerism between CD45.1 recipient cells and CD45.2 donor cells. (d) Graphical representation of the chimerism in all of the experimental animals correlating the chimerism of the three peritoneal MØ subsets with that of Ly-6Chighblood monocytes within the same animal. Data were analysed by linear regression, andr2values are indicated alongside significance testing for a non-zero slope. Each symbol represents an individual irradiation chimera. Figure 2: Both Ly-6B + and Ly-6B − inflammatory macrophages (MØ) are derived from the bone marrow. Partial BM chimeras were generated as previously described [26] , after shielding the peritoneal cavity, and then were left to recover for 6 weeks. ( a ) Analysis of blood myeloid cell chimerism 1 day before induction of peritonitis shows a stable chimerism in all experimental animals. Each line links the data from an individual mouse. ( b ) Gating strategy for the identification of Res and inflammatory (Inf) MØ (both Ly-6B + and Ly-6B − ) 72 h after the induction of peritonitis by i.p. administration of 2 × 10 6 zymosan particles. The plot has been pre-gated on CD11b high F4/80 low-high cells as previously reported [18] . ( c ) Representative flow-cytometric analysis of the indicated MØ subsets to determine the level of chimerism between CD45.1 recipient cells and CD45.2 donor cells. ( d ) Graphical representation of the chimerism in all of the experimental animals correlating the chimerism of the three peritoneal MØ subsets with that of Ly-6C high blood monocytes within the same animal. Data were analysed by linear regression, and r 2 values are indicated alongside significance testing for a non-zero slope. Each symbol represents an individual irradiation chimera. Full size image The Ly-6B + subset of inflammatory macrophages proliferate Recent murine and human studies have highlighted the selective proliferative expansion of Res macrophages, microglia and Langerhans cells during development, helminth infection and following recovery from acute inflammation [18] , [20] , [21] , [22] , [23] , [26] . Previously, we showed minimal evidence for inflammatory macrophage proliferation during inflammation [18] . To determine if a specific subset of inflammatory macrophages were proliferating within an inflammatory lesion, we adopted definitive measures of macrophage proliferation [18] to identify cells in the S, G2 and M phases of cell cycle, and also those in active cell division (phospho-Histone H3 (pHH3)-positive cells with 4N DNA content; Fig. 3 ). We found that proliferating macrophages were markedly enriched in the Ly-6B-expressing subset ( Fig. 3a ). Similarly, Ly-6B + inflammatory macrophages were also preferentially proliferating at this time in the high-dose zymosan (2 × 10 7 particles) challenge model ( Supplementary Fig. S1a,b ). 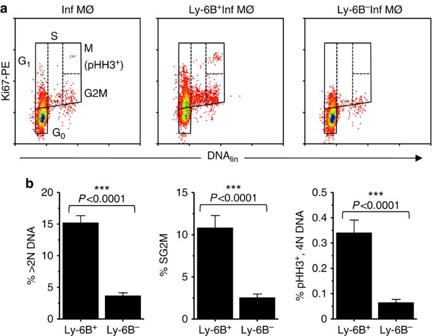Figure 3: Ly-6B-expressing inflammatory macrophages (MØ) actively dividein situ. (a) The plots show total inflammatory (Inf) MØ populations (left), Ly-6B+cells (middle) and their Ly-6B−counterparts (right) 72 h after the induction of peritonitis with 2 × 106zymosan particles. As previously reported, there is only limited evidence of proliferation in the total Inf MØ population (left and Davieset al.18). However, when subdivided based on Ly-6B expression there was a clear enrichment of cells in the S, G2 and M stages of cell cycle amongst the Ly-6B-expressing cells (middle) and notable lack of proliferating cells within the Ly-6B−population (right). Data are derived from individual mice and are representative of at least 3 experiments with 6- to 7-week-old C57BL/6 female mice and typically 3–5 mice per experiment. (b) The levels of proliferation within the two populations of Inf MØ in the same experiment shown above (a) was measured by the proportion of cells with >2N DNA content (left), >2N DNA content with Ki67 expression (‘SG2/M’, middle), phospho-Histone H3+phase of mitosis (‘pHH3+’; right). Data are expressed as mean±s.e.m. of 5 mice per group (7-week-old female C57BL/6) and is representative of at least three experiments. Data were analysed by a pairedt-test, ***P<0.001. Figure 3: Ly-6B-expressing inflammatory macrophages (MØ) actively divide in situ . ( a ) The plots show total inflammatory (Inf) MØ populations (left), Ly-6B + cells (middle) and their Ly-6B − counterparts (right) 72 h after the induction of peritonitis with 2 × 10 6 zymosan particles. As previously reported, there is only limited evidence of proliferation in the total Inf MØ population (left and Davies et al. [18] ). However, when subdivided based on Ly-6B expression there was a clear enrichment of cells in the S, G2 and M stages of cell cycle amongst the Ly-6B-expressing cells (middle) and notable lack of proliferating cells within the Ly-6B − population (right). Data are derived from individual mice and are representative of at least 3 experiments with 6- to 7-week-old C57BL/6 female mice and typically 3–5 mice per experiment. ( b ) The levels of proliferation within the two populations of Inf MØ in the same experiment shown above ( a ) was measured by the proportion of cells with >2N DNA content (left), >2N DNA content with Ki67 expression (‘SG2/M’, middle), phospho-Histone H3 + phase of mitosis (‘pHH3 + ’; right). Data are expressed as mean±s.e.m. of 5 mice per group (7-week-old female C57BL/6) and is representative of at least three experiments. Data were analysed by a paired t -test, *** P <0.001. Full size image We compared zymosan peritonitis with thioglycollate broth-induced peritonitis. This comparison is interesting because thioglycollate broth recruits substantial numbers of macrophages and is widely used to harvest macrophages from mice. Thioglycollate-induced peritonitis is characterized by accumulation and retention of macrophages [27] , which is reflected in the lack of detectable proliferating cells at commonly used time points [26] . As already noted ( Fig. 1 ), ‘thioglycollate macrophages’ present at 72 h post-injection were predominantly inflammatory, not Res, macrophages and Ly-6B-expressing macrophages were absent. As thioglycollate peritonitis at this time seemed to be slower to resolve (as evidenced by the lack of a restoring Res macrophage population), we examined later time points to capture evidence of resolution of inflammation ( Supplementary Fig. S1c,d ). At later time points (>7 days after intraperitoneal thioglycollate broth), both Res and Ly-6B + inflammatory macrophages were now evident and actively proliferating. Macrophage proliferation in inflammation depends on M-CSF We have previously shown that Res macrophage can self-renew by local proliferation [18] . Having demonstrated that a subset of BM-derived inflammatory macrophages also proliferates during inflammation, we have identified that two distinct lineages of macrophages are proliferating at specific stages within an inflammatory response. To identify the factors governing their turnover, we first examined the importance of M-CSF, a monocytic differentiation/survival factor, which is detectable at substantial levels in the peritoneal cavity of both naïve and inflammatory-challenged mice ( Supplementary Fig. S2 ). First, we tested whether elevated levels of M-CSF were sufficient to induce the expansion of Res macrophage ( Fig. 4 ). Naïve mice received 0.4 μg (i.p.) of recombinant M-CSF (Peprotec) or carrier alone ( Fig. 4a ). M-CSF dosing caused only a mild increase in Res macrophage proliferation above that obtained by injection of carrier ( Fig. 4a ). Next, to determine if M-CSF was required for proliferation of macrophage during inflammation, mice were injected with 2 × 10 6 zymosan particles in conjunction with 0.5 mg of anti-M-CSF (clone 5A1) or IgG1 control antibody. After 48 h, when Res macrophage proliferation was maximal, cells were recovered and analysed by flow cytometry. Blockade of M-CSF caused a total abrogation of Res macrophage proliferation ( Fig. 4b ). Although Ki67 is a good indicator of proliferative potential and a measure of G 1 in these macrophages (Davies et al. [18] and this study), it is a poor indicator of active cell division ( Supplementary Fig. S3 ). However, the impact of M-CSF neutralization was evident across all measures of cell cycle. 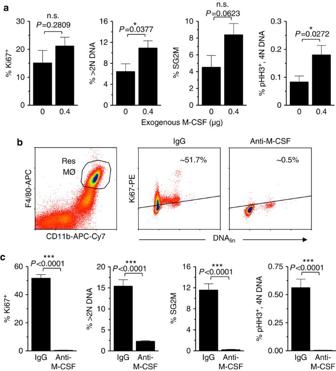Figure 4: M-CSF is required for tissue-resident macrophage proliferation. (a) Data showing proliferation of Res MØ (gated by their F4/80highCD11bhighphenotype), 24 h after i.p. administration of 0.4 μg of recombinant M-CSF (0.4) or carrier control (0). Data shown represent mean±s.e.m. 10 mice per group (7-week-old female C57BL/6) pooled from two identical experiments. Data were analysed by a Student’st-test. (b) Representative flow-cytometric plots showing the identification of Res MØ in a similar way as previously described 48 h after the i.p. injection of 2 × 106zymosan particles in conjunction with 0.5 mg of either anti-M-CSF (clone 5A1) or and rat IgG isotype control (as indicated). Percentages shown are mean values from the analyses of groups of mice (shown below). (c) Measurement of proliferation in Res MØ 48 h after i.p. injection of 2 × 106zymosan particles in conjunction with 0.5 mg of either anti-M-CSF (clone 5A1) or and rat IgG isotype control. Data shown represent mean±s.e.m. 5 mice per group (7-week-old female C57BL/6) from one of two similar experiments. Data were analyzed by a Student’st-test, *P<0.05, ***P<0.001. Figure 4: M-CSF is required for tissue-resident macrophage proliferation. ( a ) Data showing proliferation of Res MØ (gated by their F4/80 high CD11b high phenotype), 24 h after i.p. administration of 0.4 μg of recombinant M-CSF (0.4) or carrier control (0). Data shown represent mean±s.e.m. 10 mice per group (7-week-old female C57BL/6) pooled from two identical experiments. Data were analysed by a Student’s t -test. ( b ) Representative flow-cytometric plots showing the identification of Res MØ in a similar way as previously described 48 h after the i.p. injection of 2 × 10 6 zymosan particles in conjunction with 0.5 mg of either anti-M-CSF (clone 5A1) or and rat IgG isotype control (as indicated). Percentages shown are mean values from the analyses of groups of mice (shown below). ( c ) Measurement of proliferation in Res MØ 48 h after i.p. injection of 2 × 10 6 zymosan particles in conjunction with 0.5 mg of either anti-M-CSF (clone 5A1) or and rat IgG isotype control. Data shown represent mean±s.e.m. 5 mice per group (7-week-old female C57BL/6) from one of two similar experiments. Data were analyzed by a Student’s t -test, * P <0.05, *** P <0.001. Full size image When inflammatory macrophage were examined 48 h after induction of zymosan peritonitis M-CSF was also found to be important ( Fig. 5 ). Here M-CSF neutralization led to a dramatic loss of the Ly-6B + inflammatory macrophage, which was more marked than the impact of this treatment on the inflammatory macrophage population as a whole ( Fig. 5 ). Similar results were obtained in two distinct genetic backgrounds (129S6 and C57BL/6; Fig. 5 ). 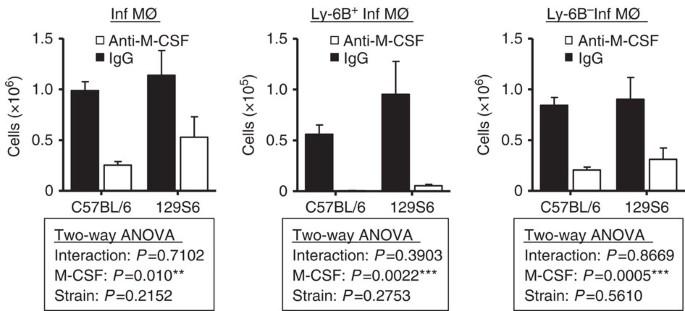Figure 5: Ly-6B-expressing inflammatory macrophages (MØ) are M-CSF-dependent. Inflammatory (Inf) MØ were quantified 48 h after acute peritonitis induced with 2 × 106zymosan particles in conjunction with 0.5 mg of either anti-M-CSF (clone 5A1) or and rat IgG isotype control. Neutralization of M-CSF results in a substantial drop in total Inf MØ numbers (left), which is caused by a near complete loss of Ly-6B+Inf MØ (middle) and substantial drop in Ly-6B−Inf MØ (right). Data shown represent mean±s.e.m. of two independent experiments conducted with 7- to 8-week-old female C57BL/6 mice (n=5 per group) and one with 9- to 12-week-old female 129S6/SvEv (n=3–6 per group). Data were analysed by two-way ANOVA with the significance of the effects of both M-CSF and strain of mouse indicated. Figure 5: Ly-6B-expressing inflammatory macrophages (MØ) are M-CSF-dependent. Inflammatory (Inf) MØ were quantified 48 h after acute peritonitis induced with 2 × 10 6 zymosan particles in conjunction with 0.5 mg of either anti-M-CSF (clone 5A1) or and rat IgG isotype control. Neutralization of M-CSF results in a substantial drop in total Inf MØ numbers (left), which is caused by a near complete loss of Ly-6B + Inf MØ (middle) and substantial drop in Ly-6B − Inf MØ (right). Data shown represent mean±s.e.m. of two independent experiments conducted with 7- to 8-week-old female C57BL/6 mice ( n =5 per group) and one with 9- to 12-week-old female 129S6/SvEv ( n =3–6 per group). Data were analysed by two-way ANOVA with the significance of the effects of both M-CSF and strain of mouse indicated. Full size image IL-4Rα is not required for macrophage proliferation Lastly, given the recently identified role for IL-4 in the selective expansion of Res macrophage in a Th2-dominated helminth infection model [26] , we examined the role of IL-4:IL-4Rα in the proliferation of Res and Ly-6B + inflammatory macrophage during acute inflammation. Mice were injected (i.p.) with 0.5 mg of anti-IL-4-neutralizing antibody (clone 11B11) or control IgG at the same time as 2 × 10 6 zymosan particles and the proliferative state of Res macrophage was analysed 48 h later. Data for cells in the definitive S, G2 or M phases of cell cycle ( Fig. 6a , left panel) and pHH3 + mitotic phases (right panel) showed no differences in the proportions of Res macrophage proliferating ( Fig. 6a ). Similar results were obtained in two genetic backgrounds (129S6 and C57BL/6; Fig. 6a ). 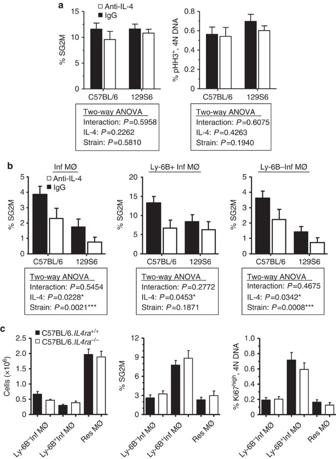Figure 6: Lack of an essential role for IL-4/IL-4Rα for macrophage (MØ) proliferation during acute inflammation. (a) Measurement of proliferation in Res MØ 48 h after i.p. injection of 2 × 106zymosan particles in conjunction with 0.5 mg of either anti-IL-4 (clone 11B11) or and rat IgG isotype control. The left graph shows the proportion of Res MØ in the S, G2 and M phases of cell cycle, whereas the right graph shows those cells in pHH3+-definitive stages of mitosis. (b) Analysis of proliferation of inflammatory (Inf) MØ subsets in mice injected i.p. 48 h earlier with 2 × 106zymosan particles in conjunction with 0.5 mg of either anti-IL-4 (clone 11B11) or and rat IgG isotype control. Data shown for panelsaandbrepresent mean±s.e.m. from two independent experiments (7-week-old female C57BL/6n=5 mice per group, and 6- to 9-week-old female 129S6 micen=3–6 mice per group). Data were analysed by a two-way ANOVA with the significance of the effects of IL-4 neutralization and mouse strain indicated. (c) The number and proliferation of the Res and Inf MØ subsets were examined 72 h after induction of peritonitis with 2 × 106zymosan particles in wild type and IL-4Rα-deficient mice on the C57BL/6 background. Data shown represent mean±s.e.m. of 6-week-old female mice (n=10 per group). Figure 6: Lack of an essential role for IL-4/IL-4Rα for macrophage (MØ) proliferation during acute inflammation. ( a ) Measurement of proliferation in Res MØ 48 h after i.p. injection of 2 × 10 6 zymosan particles in conjunction with 0.5 mg of either anti-IL-4 (clone 11B11) or and rat IgG isotype control. The left graph shows the proportion of Res MØ in the S, G2 and M phases of cell cycle, whereas the right graph shows those cells in pHH3 + -definitive stages of mitosis. ( b ) Analysis of proliferation of inflammatory (Inf) MØ subsets in mice injected i.p. 48 h earlier with 2 × 10 6 zymosan particles in conjunction with 0.5 mg of either anti-IL-4 (clone 11B11) or and rat IgG isotype control. Data shown for panels a and b represent mean±s.e.m. from two independent experiments (7-week-old female C57BL/6 n =5 mice per group, and 6- to 9-week-old female 129S6 mice n =3–6 mice per group). Data were analysed by a two-way ANOVA with the significance of the effects of IL-4 neutralization and mouse strain indicated. ( c ) The number and proliferation of the Res and Inf MØ subsets were examined 72 h after induction of peritonitis with 2 × 10 6 zymosan particles in wild type and IL-4Rα-deficient mice on the C57BL/6 background. Data shown represent mean±s.e.m. of 6-week-old female mice ( n =10 per group). Full size image Examination of the inflammatory macrophage present at this time demonstrated a partial reduction in the proliferation of these cells after neutralization of IL-4 in two independent experiments with different strains of mice ( Fig. 6b ). However, examination of the proliferation of Res and inflammatory macrophage subsets in wild-type C57BL/6 and C57BL/6. Il4ra −/− backcrossed mice, 72 h after induction of zymosan peritonitis resulted in a failure to observe any differences in either the number of cells present ( Fig. 6c , left panel) or the occurrence of proliferating cells in either of the Res or inflammatory macrophage subsets ( Fig. 6c , middle and right panels). Tissue macrophages are traditionally viewed as terminally differentiated populations, lacking in significant proliferative capacity. This view is however changing, and several murine studies have highlighted the selective proliferative expansion of Res macrophage, microglia and Langerhans cells during development, helminth infection and following recovery from acute inflammation [18] , [20] , [21] , [22] , [23] , [26] . Comparable human studies also describe proliferation of Langerhans cells [21] (and reviewed in Chorro and Geissmann [20] ), macrophages in glomerulonephritis [28] , [29] and atherosclerosis [30] and of a human monocyte subpopulation in vitro [31] . Treatment of human monocytes with M-CSF also induces genes involved in cell cycle [32] . While these studies provide a potential link between macrophage proliferation and human pathology, a clear demonstration of the proliferation of monocyte-derived macrophages in the physiological inflammatory environment in vivo has not been described. We have now specifically identified a subset of proliferating BM-derived macrophages. These cells are a quite distinct lineage branch from that of Res macrophages, which also proliferate as a mechanism of self-renewal in the tissue [18] . This separation in origins was confirmed by adoptive transfer with CD45 allotype mismatched cells [18] . However, the proliferative capacity of both subsets appears to be independently controlled. Ly-6B + inflammatory macrophages retained a capacity to undergo proliferation at a stage of acute inflammation when Res macrophage no longer exhibited significant levels of cell division [18] . The proliferation of Ly-6B + inflammatory macrophage was confirmed with definitive quantification of mitosis. We next sought to define the signals that govern macrophage proliferation. In this respect, we show an absolute requirement for M-CSF. Not only is M-CSF fundamental for Res macrophage proliferation during the proliferative burst [18] seen during the resolution of inflammation, but also basally during homoeostasis, as determined with neutralizing antibody treatment of naïve mice (not shown). Indeed, mice deficient in M-CSF due to a naturally occurring mutation (the osteopetrotic ( op/op ) mice) display a marked deficiency in many macrophage populations [33] , [34] . This suggests little role for IL-34 in this model, which would be consistent with its tissue-restricted function [35] . In spite of this, administration of additional exogenous M-CSF had only limited, albeit significant, impact on the proliferation of Res macrophages indicating that while necessary for proliferation (as demonstrated with the M-CSF neutralization experiments), it was not sufficient to cause a substantial increase in Res macrophage proliferation. In addition, inflammatory macrophage numbers were reduced in all subsets following M-CSF neutralization, suggesting that M-CSF is necessary for the normal recruitment/differentiation/survival/proliferation of inflammatory macrophage. This is particularly evident within Ly-6B + inflammatory macrophages. Thus, M-CSF is essential for maintenance of two distinct lineage branches of proliferating macrophages. When adoptively transferred into zymosan peritonitis, Ly-6B + inflammatory macrophages persisted well with 75% of the transferred number of cells still present 90 h later ( Supplementary Fig. S4 ). These cells exhibited reduced Ly-6B expression indicating that Ly-6B + inflammatory macrophages may become Ly-6B − inflammatory macrophages ( Supplementary Fig. S4 ). Recently, IL-4 was identified as important for the expansion of Res macrophage during helminth infection [26] . While IL-4-driven macrophage proliferation is consistent with a role during Th2 immunity, its role in other inflammatory settings has not been determined. Our data using both IL-4 neutralizing antibody and Il4ra −/− mice demonstrate that IL-4Rα is not essential for the proliferation of either Res or inflammatory macrophage subsets in acute inflammation, although we cannot exclude that IL-4 has a more limited role as a modulator of inflammatory macrophage proliferation. The lack of a requirement for IL-4Rα in this innate inflammatory model suggests that IL-4-driven proliferation is restricted to Th2 settings. Indeed, in helminth infection models, IL-4-dependent macrophage accumulation does not occur in the absence of Th2 cells [36] , suggesting that innate sources of IL-4 are not sufficient to drive proliferation. Critically, these observations indicate that macrophage proliferation is a general phenomenon that is not restricted to IL-4 and Th2 immunity. Our findings indicate that both Res macrophages and inflammatory macrophage are capable of proliferating during key stages of the inflammatory response. While proliferating inflammatory macrophages are found throughout the resolution phase of inflammation, Res macrophage proliferation appears to be tightly governed and is restricted once normal tissue numbers are restored [18] . Res macrophages and Ly-6B + inflammatory macrophages are therefore likely to potentiate unique biological activities. Re-establishment of the tissue-resident population and continued presence of an inflammatory cell involved in pathogen or injury control are highly distinct functions and yet both require M-CSF. Considering the extensive development of M-CSF as therapeutic target [37] , understanding these dynamics is essential and illustrates the need to unravel the contribution of macrophage origins to eventual function. It will be interesting to determine whether these findings within the peritoneal cavity applies to other tissues. In this context, Yona et al. [38] recently demonstrated that the relative autonomy of tissue-resident macrophages, which we have reported in the serosal cavities [18] , [26] appears to be widespread. The proliferation of inflammatory macrophages in other contexts, while likely to occur, would need to be addressed in each context. In summary, our data demonstrate that proliferation provides a general mechanism for the expansion of both peripherally derived (inflammatory) and Res macrophage lineages during the resolution of inflammation. This raises critical new questions about the contribution of proliferation versus recruitment to monocyte/macrophage function and the different roles of macrophage subsets. For example, does the failure of a particular subset to proliferate contribute to chronic inflammatory pathology, or does excessive proliferation promote unwanted tissue repair and fibrosis? The answers to these questions will open new avenues for understanding the optimal immune responses and intervention strategies required for the restoration of normal tissue homoeostasis. Mice C57BL/6 female mice were obtained from Harlan Olac and 129S6/SvEv mice from our own breeding colonies and were used between 6–7 weeks of age (unless otherwise stated). C57BL/6. Il4ra −/− mice were generated by backcrossing Il4ra −/− (ref. 39 ) onto the C57BL/6 genetic background for at least nine generations. Peritonitis was induced typically by i.p. injection of 2 × 10 6 (unless otherwise indicated) zymosan particles in 100 μl of PBS or with 1 ml of 4% Brewer’s thioglycollate medium (Sigma, B2551). For antibody modulation experiments, 0.5 mg of anti-M-CSF (clone 5A1), anti-IL-4 (clone 11B11) or control IgG were co-injected with the zymosan in a total volume of 250 μl of PBS. Exogenous M-CSF (Peprotec) was administered i.p. in 250 μl total volume in a solution of 0.05% BSA in PBS and control mice received this vehicle alone. Peritoneal cells were recovered at the indicated time points after killing of the animal by lavage with 5 ml of ice-cold 5 mM EDTA in PBS and absolute cell counts were determined using a hemacoytometer before further analysis. All animal work was conducted in line with Institutional and UK Home Office guidelines. Partial BM chimeras were generated by shielding the peritoneal cavity and irradiation, as previously described [26] . Antibodies and immunoassays Antibodies used were: anti-Ly-6B.2-phycoerythrin (PE) or –A647 (clone 7/4 (ref. 6 ); AbD Serotec); anti-Ly-6B.2-Peridinin-chlorophyll-protein (PerCP) (clone 7/4 labelled using the Phycolink PerCP-labeling kit from Europa Bioproducts); anti-Ly-6G-PE-Cy7 (clone 1A8; BD Biosciences); anti-CD11b-APC or -APC-Cy7 or PerCP-Cy5.5 (clone M1/70; BD Biosciences); anti-CD11b-FITC (clone 56C; homemade); anti-Tim4-PE (clone RMT4-54; eBiosciences); anti-F4/80-PE or -Alexa405 or -APC (clone CL:A3-1; AbD Serotec); anti-F4/80-PE-Cy7 (Biolegend) or -PE-Texas Red (PE-TxR) (clone BM8; Invitrogen); anti-Ki67-PE (clone B56) and IgG1κ-PE (clone MOPC-21; BD Biosciences); anti-pHH3-A488 (clone D2C8 (Ser10); New England Biolabs); anti-CD45.1-FITC (clone A20; Biolegend); anti-CD45.2-APC-Cy7 (clone 104; Biolegend); Streptavidin-PE-TxR and steptavidin-PerCP was obtained from BD Biosciences. The supplier for 4′,6-diamidino-2-phenylindole (DAPI) was Invitrogen. M-CSF in lavage fluid was measured using the mouse M-CSF ELISA kit (Peprotec) as directed by the manufacturer. Flow cytometry and flow-cytometric cell sorting Flow-cytometric staining was conducted using the standard protocols in our laboratory [6] , [12] , [18] , [25] . For cell purification, lavage from mice 7 days after induction of peritonitis with 2 × 10 6 zymosan particles were pooled, stained as indicated in Figure 1e and sorted on a MoFlo Legend (Beckman-Coulter) for single events (via pulse width) with the defined flow-cytometric phenotype and appropriate FSC/SSC profiles (see Fig. 1 and Taylor et al. [6] , [12] , [18] ). The purity of the sorted populations was verified after sorting and morphology was investigated on cytospin preparations, which were stained and visualized using Microscopy Hemacolour cell stain (Merck). Analytical polychromatic flow cytometry was conducted on a CyAn ADP analyzer (Beckman-Coulter) and analysed using Summit software v4.3 (Beckman-Coulter) or on a Canto II (BD) and analysed using FlowJo (TreeStar) and when appropriate was related to the absolute cell counts of the individual animals. Statistical analysis Two-way ANOVAs, Student’s t -tests (paired or unpaired) and linear regression analysis were conducted using GraphPad Prism and the tests and results are indicated in the appropriate text. Statistical significance is also highlighted with the following notations: * P <0.05; ** P <0.01; *** P <0.001. How to cite this article: Davies, L.C. et al. Distinct bone marrow-derived and tissue-resident macrophage lineages proliferate at key stages during inflammation. Nat. Commun. 4:1886 doi: 10.1038/ncomms2877 (2013).